Engineered pairs of distinct photoswitches for optogenetic control of cellular proteins Optogenetic methods take advantage of photoswitches to control the activity of cellular proteins. Here, we completed a multi-directional engineering of the fungal photoreceptor Vivid to develop pairs of distinct photoswitches named Magnets. These new photoswitches were engineered to recognize each other based on the electrostatic interactions, thus preventing homodimerization and enhancing light-induced heterodimerization. Furthermore, we tuned the switch-off kinetics by four orders of magnitude and developed several variants, including those with substantially faster kinetics than any of the other conventional dimerization-based blue spectrum photoswitches. We demonstrate the utility of Magnets as powerful tools that can optogenetically manipulate molecular processes in biological systems. Several natural photoreceptors derived from plants, fungi and bacteria, such as the LOV2 domain of phototropin 1, phytochrome B, cryptochrome 2 (CRY2), FKF1, Vivid (VVD), UVR8 and EL222, have been used as photoswitches to construct the optogenetic tool known as a photoactivatable actuator [1] , [2] , [3] , [4] , [5] , [6] , [7] , [8] , [9] , [10] . These photoreceptor-based photoswitches proved that the methods used to control protein activities with light provide a powerful approach to perturbing cellular signalling processes, such as cell morphology [4] , [5] , [6] , signal transduction [5] and gene expression [2] , [3] , [6] , [7] , [8] , [9] , [10] . In addition to the photoswitches developed from natural photoreceptors, engineered photoswitches (TULIPs, LOV-ipaA and LOV-SsrA) based on peptide-tagged LOV2 domains and peptide-binding domains/proteins have been recently developed [11] , [12] . Here, we describe novel photoswitches made from the multi-directional engineering of a blue light photoreceptor VVD derived from the filamentous fungus Neurospora crassa [13] . VVD is currently one of the smallest photoreceptors among those tested as optogenetic tools, and its cofactor is flavin adenine dinucleotide, which is abundant in eukaryotic cells. In addition, VVD can switch from a monomer to a homodimer in response to blue light [13] , [14] , [15] . This dynamic dimerization property of VVD is useful for controlling the protein–protein interactions. Despite the competitive advantages of VVD described above, it has several undesired properties that can be improved. For example, the homodimerization property of VVD could cause serious problems in efficiency and selectivity. In addition, the switch-off kinetics of VVD are too slow (half life t 1/2 , 2.8 h) [13] , [14] , [16] to precisely control protein activities at the subcellular level. In addition, its dimerization affinity is low [14] . Because the nature of photoswitches is directly linked to the overall performance of optogenetic tools, the development of robust and versatile photoswitches that overcome limitations of natural photoreceptors is essential to control cellular proteins with light. To address the multiple limitations of VVD, we first engineered its homodimer interface and developed two distinct types of VVD variants, which we named Magnets. The Magnet pairs are engineered to recognize each other through electrostatic interactions, thus preventing unwanted homodimerization and selectively inducing heterodimerization with light. In addition to re-engineering the dimerization property of VVD, we tuned the switch-off kinetics of the photoswitches. We developed variants with kinetics that differed by up to four orders of magnitude within the range of seconds to hours. The variants included those with substantially faster switch-off kinetics than any other existing dimerization-based blue photoswitches. In the process of tuning the switch-off kinetics, we found a key engineering approach to creating Magnet pairs with substantially improved dimerization efficiencies. Next, we demonstrated the utility of the present photoswitches by exerting spatially and temporally precise control over several signalling proteins in living mammalian cells. The present photoswitches, Magnets, offer a powerful tool for optogenetically manipulating molecular processes in biological systems and permitting a deeper understanding of living cells with high spatiotemporal precision. Design of two distinct VVD variants VVD is a small photoreceptor that reversibly switches its state from a monomer to a homodimer in response to blue light [13] , [14] , [15] ( Fig. 1a ). This dynamic dimerization property of VVD is useful; however, its homodimerization property can also cause serious problems. For example, when VVD is used as a photoswitch to bring two different proteins (protein A and protein B) close to each other, the photoreceptor induces not only the A–B interaction but also unwanted A–A and B–B interactions ( Fig. 1b ). Thus, this property prevents the efficient induction of the intended A–B interaction and can cause undesirable side effects resulting from the A–A and B–B interactions. To overcome this limitation of VVD, we first engineered its homodimer interface, termed Ncap [13] , [15] ( Fig. 1a ). The Ncap from Ile47 to Asn56 consists of neutral amino acids ( Fig. 1a ). We developed two distinct types of VVD variants: one with positively charged amino acids in the Ncap and the other with negatively charged amino acids in the Ncap ( Fig. 1c ). Unlike VVD, the two VVD variants recognized each other based on electrostatic interactions (attraction and repulsion). The two VVD variants negate the possibility that unwanted A–A and B–B interactions are induced, thereby selectively triggering the induction of the expected A–B interaction with light. 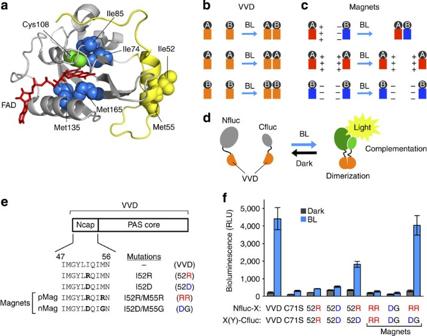Figure 1: The design and development of Magnets. (a) The Vivid (VVD) structure and its key amino acid residues. Blue light irradiation triggers the formation of a photo-adduct between Cys108 (green) and the isoalloxazine ring of flavin adenine dinucleotide (FAD; red), thus inducing VVD dimerization. The N-terminal α-helix, termed Ncap (yellow), is located at the interface of the dimer. The amino acid sequence of the Ncap from Ile47 to Asn56 consists of neutral amino acid residues (IMGYLIQIMN). Photocycle-related residues are shown in blue. (b) As a photoswitch, VVD (orange square) induces the interaction between protein A and protein B but also the unwanted A–A and B–B interactions in response to blue light. (c) These two VVD variants (red and blue squares) use electrostatic interactions to prevent homodimerization and selectively induce heterodimerization. (d) A schematic of the bioluminescence assay system that reports VVD dimerization. One VVD is tagged with a N-half fragment (Nfluc) of split-firefly luciferase, and the other VVD is tagged with the C-half fragment (Cfluc). These fusions are monomers in the dark state and have no bioluminescence activity. Upon blue light irradiation, rapid dimerization of VVD leads to the complementation of Nfluc and Cfluc and induction of bioluminescence. This assay system allows for the reversible detection of VVD dimerization. (e) Schematic representation of VVD domains and its variants. The characteristic mutations used in this study are highlighted. (f) The bioluminescence assay of VVD dimerization before and after blue light irradiation. Nfluc-X and Y(X)-Cfluc (X and Y stand for VVD variants) were coexpressed in COS-7 cells. The cells were irradiated with blue light (470±20 nm, 3 mW cm−2) for 30 s, and bioluminescence measurements of live cells were performed. The results are shown as the mean±s.d. of three independent measurements. RLU, relative light unit. Figure 1: The design and development of Magnets. ( a ) The Vivid (VVD) structure and its key amino acid residues. Blue light irradiation triggers the formation of a photo-adduct between Cys108 (green) and the isoalloxazine ring of flavin adenine dinucleotide (FAD; red), thus inducing VVD dimerization. The N-terminal α-helix, termed Ncap (yellow), is located at the interface of the dimer. The amino acid sequence of the Ncap from Ile47 to Asn56 consists of neutral amino acid residues (IMGYLIQIMN). Photocycle-related residues are shown in blue. ( b ) As a photoswitch, VVD (orange square) induces the interaction between protein A and protein B but also the unwanted A–A and B–B interactions in response to blue light. ( c ) These two VVD variants (red and blue squares) use electrostatic interactions to prevent homodimerization and selectively induce heterodimerization. ( d ) A schematic of the bioluminescence assay system that reports VVD dimerization. One VVD is tagged with a N-half fragment (Nfluc) of split-firefly luciferase, and the other VVD is tagged with the C-half fragment (Cfluc). These fusions are monomers in the dark state and have no bioluminescence activity. Upon blue light irradiation, rapid dimerization of VVD leads to the complementation of Nfluc and Cfluc and induction of bioluminescence. This assay system allows for the reversible detection of VVD dimerization. ( e ) Schematic representation of VVD domains and its variants. The characteristic mutations used in this study are highlighted. ( f ) The bioluminescence assay of VVD dimerization before and after blue light irradiation. Nfluc-X and Y(X)-Cfluc (X and Y stand for VVD variants) were coexpressed in COS-7 cells. The cells were irradiated with blue light (470±20 nm, 3 mW cm −2 ) for 30 s, and bioluminescence measurements of live cells were performed. The results are shown as the mean±s.d. of three independent measurements. RLU, relative light unit. Full size image Development of Magnets To monitor the blue light-dependent dimerization of VVD and its variants, we developed a bioluminescence assay system based on the complementation of split-firefly luciferase fragments [17] ( Fig. 1d and Supplementary Figs 1 and 2 ). Using this system, we systematically searched for key amino acid residues in the Ncap of VVD that would lead to the expected electrostatic discrimination once substituted ( Fig. 1e and Supplementary Fig. 3 ). We individually substituted each amino acid residue from 47 to 56 in the Ncap with a negatively charged amino acid and identified variants that showed impaired homodimerization because of electrostatic repulsion ( Supplementary Fig. 3a ). We found that the single substitution of Ile52 with aspartic acid substantially decreased the blue light-dependent homodimerization of the VVD variant to similar levels observed in the nonfunctional VVD-C71S variant [13] ( Fig. 1f and Supplementary Fig. 3f,g ). We also substituted amino acid residue 52 of VVD with a positively charged amino acid and showed that an arginine substitution effectively suppressed the homodimerization of the VVD variant ( Fig. 1f and Supplementary Fig. 3f,g ). Next, we examined the heterodimerization of the I52R and I52D variants and found that these two variants showed a significant bioluminescence response upon blue light irradiation ( Fig. 1f and Supplementary Fig. 3f,g ). This result indicates that the I52R and I52D substitutions efficiently induced heterodimerization and suppressed homodimerization of the VVD variants. Using mutagenesis of Met55 within both I52R and I52D variants showed that I52R/M55R and I52D/M55G variants were more effective at promoting heterodimerization than other variants ( Fig. 1f and Supplementary Fig. 3l ). The blue light-dependent heterodimerization of I52R/M55R and I52D/M55G variants was largely improved (light/dark, 21-fold) when compared with the I52R and I52D variants (light/dark, 6.0-fold). In addition, I52R/M55R and I52D/M55G variants were more effective at preventing homodimerization when compared with the I52R and I52D variants, respectively ( Fig. 1f and Supplementary Fig. 3m,h ). As a result of the double substitutions at residues 52 and 55, the pair of I52R/M55R and I52D/M55G variants were selected as the top pair of distinct VVD variants that recognize each other based on electrostatic interactions ( Fig. 1e ). On the basis of their electrostatic interactions, the VVD variants were collectively named ‘Magnets’. Specifically, the I52R/M55R variant has a positively charged arginine at residue 52 and was named ‘positive Magnet (pMag)’, and I52D/M55G has a negatively charged aspartic acid at residue 52 and was named ‘negative Magnet (nMag)’. Tuning switch-off kinetics and dimerization efficiencies pMag and nMag quickly form a heterodimer upon blue light irradiation; however, it takes hours for the complex to dissociate after the blue light is shut off ( t 1/2 , 1.8 h; rate constant, 1.1 × 10 −4 ; Fig. 2a ). The slow switch-off kinetics of the pMag–nMag complex is similar to that of the homodimer of VVD ( t 1/2 , 2.0 h; rate constant, 9.5 × 10 −5 ; Supplementary Fig. 4 ). To tune the switch-off kinetics, we added mutations to Ile74, Ile85, Met135 and Met165 within the Per-Arnt-Sim (PAS) core of both pMag and nMag because these changes were reported to shorten or lengthen the photocycle of VVD [16] ( Fig. 2b ). The substitution of Ile85 with valine in both pMag and nMag caused the complex of the two variants to dissociate with half-life t 1/2 of 4.2 min (rate constant, 2.7 × 10 −3 ), which is 25-fold faster than the pMag–nMag complex ( Fig. 2a ); thus, we renamed the two variants pMagFast1 and nMagFast1. Another set of two variants with substitutions of both Ile74 and Ile85 with valine exhibited a substantially accelerated dissociation ( t 1/2 , 25 s; rate constant, 2.8 × 10 −2 ) that was 250-fold faster than the pMag–nMag complex ( Fig. 2a ). The two variants were named pMagFast2 and nMagFast2. Therefore, substitutions that shorten the photocycle reduce the time needed for the dissociation of the pMag and nMag complexes. 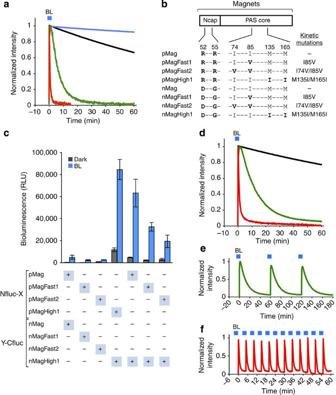Figure 2: Tuning of the dissociation kinetics and dimerization efficiency of the photoswitches. (a) Dissociation kinetics of pMag–nMag (black), pMagFast1–nMagFast1 (green), pMagFast2–nMagFast2 (red) and pMagHigh1–nMagHigh1 (blue). COS-7 cells co-expressing Nfluc-X and Y-Cfluc (X and Y stand for pMag variants and nMag variants, respectively) were irradiated with blue light at time 0 for 30 s to induce complex formation prior to observing the dissociation of the present photoswitches. (b) Schematic representation of the variants with kinetic mutations within the Per-Arnt-Sim (PAS) core. (c) Changing the photocycle substantially affects the extent of dimerization of the photoswitches after blue light irradiation. The results are shown as the mean±s.d. of three independent measurements. (d) Dissociation kinetics of pMagFast1–nMagHigh1 (green), pMagFast2–nMagHigh1 (red) and pMag–nMagHigh1 (black). (e,f) Reversible and repeatable dimerization and dissociation properties of pMagFast1–nMagHigh1 (e) and pMagFast2–nMagHigh1 (f). The resultsaandd–frepresent typical experiments from three independent measurements. Figure 2: Tuning of the dissociation kinetics and dimerization efficiency of the photoswitches. ( a ) Dissociation kinetics of pMag–nMag (black), pMagFast1–nMagFast1 (green), pMagFast2–nMagFast2 (red) and pMagHigh1–nMagHigh1 (blue). COS-7 cells co-expressing Nfluc-X and Y-Cfluc (X and Y stand for pMag variants and nMag variants, respectively) were irradiated with blue light at time 0 for 30 s to induce complex formation prior to observing the dissociation of the present photoswitches. ( b ) Schematic representation of the variants with kinetic mutations within the Per-Arnt-Sim (PAS) core. ( c ) Changing the photocycle substantially affects the extent of dimerization of the photoswitches after blue light irradiation. The results are shown as the mean±s.d. of three independent measurements. ( d ) Dissociation kinetics of pMagFast1–nMagHigh1 (green), pMagFast2–nMagHigh1 (red) and pMag–nMagHigh1 (black). ( e , f ) Reversible and repeatable dimerization and dissociation properties of pMagFast1–nMagHigh1 ( e ) and pMagFast2–nMagHigh1 ( f ). The results a and d – f represent typical experiments from three independent measurements. Full size image Despite the successful tuning of the switch-off kinetics of the pMag–nMag complex, we noticed that the bioluminescence signals after the dimerization of pMagFast1 with nMagFast1 and pMagFast2 with nMagFast2 decreased to 47% and 51% of pMag and nMag, respectively ( Fig. 2c and Supplementary Fig. 5 ). The result shows that a change in the photocycles of pMag and nMag substantially affected the extent of dimerization and revealed an undesirable functional correlation between fast dissociation kinetics and dimerization efficiency. This unwanted trade-off is an unacceptable limitation in the development of useful photoswitches. To overcome this problem, we focused on other photocycle-related substitutions. M135I and M165I substitutions can lengthen the photocycle of VVD [16] and substantially decelerate the dissociation of the pMag–nMag complex ( t 1/2 , 4.7 h; rate constant, 4.1 × 10 −5 ; Fig. 2a ). We found that these two substitutions dramatically increased the extent of light-dependent dimerization of pMag and nMag up to 1,700% ( Fig. 2c and Supplementary Fig. 5 ). The pMag and nMag variants were named pMagHigh1 and nMagHigh1, respectively. We examined the blue light-dependent heterodimerization between pMag variants and nMag variants with different switch-off kinetics. The extent of heterodimerization of pMagFast1 and nMagHigh1, which exhibited fast and slow switch-off kinetics, respectively, was enhanced up to 1,400% compared with pMagFast1 and nMagFast1 ( Fig. 2c ). The combination of pMagFast2 and nMagHigh1 showed an enhancement of up to 760% compared with pMagFast2 and nMagFast2 ( Fig. 2c ). The result indicates that a pairing with nMagHigh1 substantially enhanced the dimerization efficiencies of the pMag variants with fast dissociation kinetics. Furthermore, nMagHigh1 does not slow the switch-off kinetics of its heterodimers with the fast pMag variants ( Fig. 2d ). Also, pairing the fast pMag variants with nMagHigh1 did not prevent their reversible dimerization properties ( Fig. 2e,f ). In addition, the heterodimerization of pMag with nMagHigh1 was enhanced up to 1,300% without affecting the switch-off kinetics compared with pMag and nMag ( Fig. 2c,d ). Our current approach used the combination of two different kinetic variants to solve the unwanted trade-off problem and allowed us to develop photoswitches with both substantially enhanced dimerization efficiencies and accelerated switch-off kinetics. Light-dependent PM-recruitment and dissociation To further study the developed photoswitches, we added a CAAX motif (refs 18 , 19 , 20 ) to nMagHigh1 and coexpressed it with pMag-mCherry in COS-7 cells. Using total internal reflection fluorescence (TIRF) microscopy, we observed that pMag-mCherry was recruited to the plasma membrane (PM) where nMagHigh1-CAAX was tethered in a blue light-dependent manner ( Fig. 3a,b ). We also tested tandemly repeated pMag fusions ( Fig. 3b ). The apparent concentration of pMag surrounding each nMag molecule and the apparent affinity between the photoswitches were expected to increase using the tandemly repeated fusion of pMag. A two tandemly repeated pMag(2x) gave a larger TIRF response than pMag. The TIRF response was further increased using a three tandemly repeated pMag(3x), indicating that the PM-recruitment of Magnets is enhanced by using a tandemly repeated fusion. Thus, we used pMag(3x) and pMagFast2(3x) for subsequent experiments. 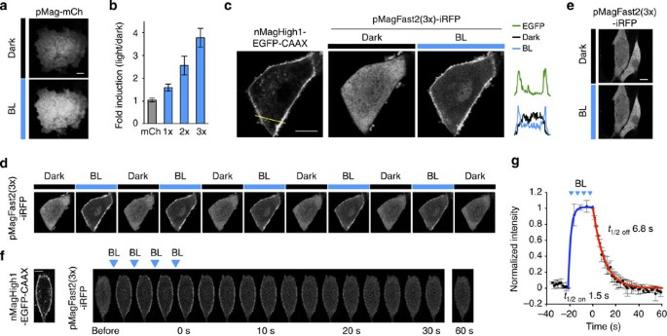Figure 3: The plasma membrane (PM)-translocation assay of the photoswitches. (a) Total internal reflection fluorescence (TIRF) microscopy images of COS-7 cells expressing pMag-mCherry before and after irradiation with evanescent light at 488 nm for 50 ms. nMagHigh1-mKikGR-CAAX is coexpressed in the cells. (b) PM-recruitment of the photoswitches after irradiation with evanescent light at 488 nm for 50 ms. mCh, mCherry; 1x, pMag-mCherry; 2x, pMag(2x)-mCherry; 3x, pMag(3x)-mCherry. The results are shown as the mean±s.d. of five independent measurements. (c) Confocal fluorescence images of a NIH3T3 cell expressing pMagFast2(3x)-iRFP and nMagHigh1-EGFP-CAAX. pMagFast2(3x)-iRFP was imaged before and after irradiation with blue light at 488 nm. Line profiles represent fluorescence intensities of EGFP (green) and iRFP (black and blue) measured along the yellow line of the nMagHigh1-EGFP-CAAX image. (d) Reversible and repeatable PM-recruitment of pMagFast2(3x)-iRFP. (e) Fluorescence images of NIH3T3 cells expressing pMagFast2(3x)-iRFP before and after blue light irradiation. (f) Time course of blue light-dependent recruitment of pMagFast2(3x)-iRFP to the PM and its dissociation to the cytosol in the dark state. PM-localization of nMagHigh1-EGFP-CAAX is shown on the left. (g) Kinetic analysis of the PM-recruitment of pMagFast2(3x)-iRFP and its dissociation to the cytosol in the dark state. The kinetic curves of the fluorescence intensity of iRFP at the PM are fitted to mono-exponential functions (on, blue; off, red). Thet1/2 on(1.5 s) andt1/2 off(6.8 s) were determined using the mono-exponential functions. The results are shown as the mean±s.d. of three independent measurements. Scale bars in all images, 10 μm. Figure 3: The plasma membrane (PM)-translocation assay of the photoswitches. ( a ) Total internal reflection fluorescence (TIRF) microscopy images of COS-7 cells expressing pMag-mCherry before and after irradiation with evanescent light at 488 nm for 50 ms. nMagHigh1-mKikGR-CAAX is coexpressed in the cells. ( b ) PM-recruitment of the photoswitches after irradiation with evanescent light at 488 nm for 50 ms. mCh, mCherry; 1x, pMag-mCherry; 2x, pMag(2x)-mCherry; 3x, pMag(3x)-mCherry. The results are shown as the mean±s.d. of five independent measurements. ( c ) Confocal fluorescence images of a NIH3T3 cell expressing pMagFast2(3x)-iRFP and nMagHigh1-EGFP-CAAX. pMagFast2(3x)-iRFP was imaged before and after irradiation with blue light at 488 nm. Line profiles represent fluorescence intensities of EGFP (green) and iRFP (black and blue) measured along the yellow line of the nMagHigh1-EGFP-CAAX image. ( d ) Reversible and repeatable PM-recruitment of pMagFast2(3x)-iRFP. ( e ) Fluorescence images of NIH3T3 cells expressing pMagFast2(3x)-iRFP before and after blue light irradiation. ( f ) Time course of blue light-dependent recruitment of pMagFast2(3x)-iRFP to the PM and its dissociation to the cytosol in the dark state. PM-localization of nMagHigh1-EGFP-CAAX is shown on the left. ( g ) Kinetic analysis of the PM-recruitment of pMagFast2(3x)-iRFP and its dissociation to the cytosol in the dark state. The kinetic curves of the fluorescence intensity of iRFP at the PM are fitted to mono-exponential functions (on, blue; off, red). The t 1/2 on (1.5 s) and t 1/2 off (6.8 s) were determined using the mono-exponential functions. The results are shown as the mean±s.d. of three independent measurements. Scale bars in all images, 10 μm. Full size image We examined the fast photoswitches consisting of pMagFast2(3x) and nMagHigh1 using confocal microscopy. Owing to the low dimerization activity of the photoswitches in the dark state, we observed no significant PM-recruitment of pMagFast2(3x)-iRFP before blue light irradiation ( Fig. 3c ). Upon irradiation with blue light, pMagFast2(3x)-iRFP was efficiently recruited to the PM where nMagHigh1-CAAX was tethered ( Fig. 3c ). When the irradiation was removed, pMagFast2(3x)-iRFP returned to the cytosol ( Fig. 3d ). The PM-recruitment of pMagFast2(3x)-iRFP was reversible and repeatable ( Fig. 3d ). We confirmed that blue light irradiation of the cells did not recruit pMagFast2(3x)-iRFP to the PM without nMagHigh1-CAAX ( Fig. 3e ). On the basis of the translocation assay, we analysed the switch-on kinetics of the fast photoswitches and showed that the PM-recruitment of pMagFast2(3x)-iRFP was rapidly induced with a t 1/2 on of 1.5 s (rate constant, 4.6 × 10 −1 ) ( Fig. 3f,g and Supplementary Movie 1 ). We also investigated switch-off kinetics and found that pMagFast2(3x)-iRFP dissociated from the PM with a t 1/2 off of 6.8 s (rate constant, 1.0 × 10 −1 ) when the blue light irradiation was removed ( Fig. 3f,g and Supplementary Movie 1 ). To our knowledge, the switch-off kinetics of the photoswitches consisting of pMagFast2(3x) and nMagHigh1 are much faster than any other dimerization-based blue photoswitches currently available [6] , [7] , [11] . Optical control of PI(3,4,5)P 3 production Next, we showed that the present photoswitches can control cellular proteins and related cellular functions. Phosphoinositides are major signalling molecules at the PM. We connected pMag(3x) with an inter-SH2 (iSH2) domain derived from a p85 regulatory subunit of phosphatidylinositol 3-kinase (PI3K). The iSH2 domain was previously paired with chemically inducible dimerizers and other blue and red light photoswitches to control PI3K activity [21] , [22] , [23] . When expressed in mammalian cells, iSH2-pMag(3x)-iRFP spontaneously binds to an endogenous p110 catalytic subunit of PI3K that generates phosphatidylinositol 3,4,5-triphosphate (PI(3,4,5)P 3 ). We coexpressed iSH2-pMag(3x)-iRFP with nMagHigh1-CAAX in NIH3T3 cells together with AktPH-mCherry, which is a PI(3,4,5)P 3 biosensor consisting of a pleckstrin homology (PH) domain [24] derived from Akt1 and mCherry. After blue light irradiation, iSH2-pMag(3x)-iRFP was immediately recruited to the PM where nMagHigh1-CAAX was tethered ( Fig. 4a ). In addition, rapid PM-recruitment of AktPH-mCherry was also observed, indicating that PI(3,4,5)P 3 was immediately produced in the PM upon blue light irradiation ( Fig. 4b ). 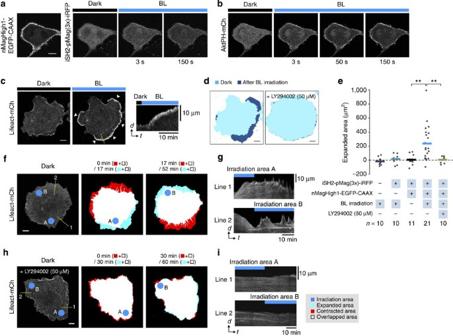Figure 4: Magnet-based photoactivatable phosphatidylinositol 3-kinase (PI3K). (a,b) Fluorescence images of a NIH3T3 cell before and after blue light irradiation. Coexpressed nMagHigh1-EGFP-CAAX (a), iSH2-pMag(3x)-iRFP (a) and AktPH-mCherry (b) were individually imaged. (c) Fluorescence images of a COS-7 cells expressing nMagHigh1-EGFP-CAAX, iSH2-pMag(3x)-iRFP and Lifeact-mCherry before and 15 min after irradiation. Arrowheads indicate lamellipodia and ruffles. The kymograph was drawn along the yellow dotted line. (d) Photoactivatable PI3K induces cell expansion. The image data incwere analysed (left). LY294002 blocked the blue light-dependent cell expansion (right). (e) Quantification of the expanded area of cells expressing photoactivatable PI3K. The expanded area was calculated by subtracting the cell area before blue light irradiation from the area after irradiation. (f) Spatiotemporally confined irradiation of a COS-7 cell expressing nMagHigh1-EGFP-CAAX, iSH2-pMagFast2(3x)-iRFP and Lifeact-mCherry. The left panel shows a fluorescence image of Lifeact-mCherry before focal irradiation. Small areas ‘A’ and ‘B’ that were sequentially irradiated at 488 nm are shown with blue circles (diameter=10 μm). Areas ‘A’ and ‘B’ were irradiated from 0 to 17 min and 17–52 min, respectively. The center panel is the merged image of the cell before and 17 min after the focal irradiation of area A. The expanded area and contracted area are shown in cyan and red, respectively. The right panel is the merged image of the cell at time points of 17 min and 52 min. (g) Kymographs were drawn along yellow dotted lines 1 and 2 shown inf. (h) The morphological changes of the cells induced by blue light were blocked by LY294002. (i) Kymographs were drawn along yellow dotted lines 1 and 2 shown inh. The resultsa–i, except fore, represent typical experiments from three independent measurements. Scale bars in all images, 10 μm. Figure 4: Magnet-based photoactivatable phosphatidylinositol 3-kinase (PI3K). ( a , b ) Fluorescence images of a NIH3T3 cell before and after blue light irradiation. Coexpressed nMagHigh1-EGFP-CAAX ( a ), iSH2-pMag(3x)-iRFP ( a ) and AktPH-mCherry ( b ) were individually imaged. ( c ) Fluorescence images of a COS-7 cells expressing nMagHigh1-EGFP-CAAX, iSH2-pMag(3x)-iRFP and Lifeact-mCherry before and 15 min after irradiation. Arrowheads indicate lamellipodia and ruffles. The kymograph was drawn along the yellow dotted line. ( d ) Photoactivatable PI3K induces cell expansion. The image data in c were analysed (left). LY294002 blocked the blue light-dependent cell expansion (right). ( e ) Quantification of the expanded area of cells expressing photoactivatable PI3K. The expanded area was calculated by subtracting the cell area before blue light irradiation from the area after irradiation. ( f ) Spatiotemporally confined irradiation of a COS-7 cell expressing nMagHigh1-EGFP-CAAX, iSH2-pMagFast2(3x)-iRFP and Lifeact-mCherry. The left panel shows a fluorescence image of Lifeact-mCherry before focal irradiation. Small areas ‘A’ and ‘B’ that were sequentially irradiated at 488 nm are shown with blue circles (diameter=10 μm). Areas ‘A’ and ‘B’ were irradiated from 0 to 17 min and 17–52 min, respectively. The center panel is the merged image of the cell before and 17 min after the focal irradiation of area A. The expanded area and contracted area are shown in cyan and red, respectively. The right panel is the merged image of the cell at time points of 17 min and 52 min. ( g ) Kymographs were drawn along yellow dotted lines 1 and 2 shown in f . ( h ) The morphological changes of the cells induced by blue light were blocked by LY294002. ( i ) Kymographs were drawn along yellow dotted lines 1 and 2 shown in h . The results a – i , except for e , represent typical experiments from three independent measurements. Scale bars in all images, 10 μm. Full size image Because PI(3,4,5)P 3 is a lipid messenger that regulates membrane morphology [25] , we examined the morphological changes in the PM of COS-7 cells that expressed iSH2-pMag(3x)-iRFP and nMagHigh1-CAAX using Lifeact-mCherry [26] . Blue light irradiation induced lamellipodia and ruffles in the PM ( Fig. 4c ). The morphological change in the PM was accompanied by actin polymerization detected with Lifeact-mCherry ( Fig. 4c and Supplementary Movie 2 ). In addition, we quantitatively analysed cell area before and after irradiation and revealed a significant blue light-dependent expansion of the cells ( Fig. 4d,e ). The observed morphological change in the PM was completely blocked by LY294002, a potent inhibitor of PI3K ( Fig. 4d,e ). We also examined cells that did not express both iSH2-pMag(3x)-iRFP and nMagHigh1-CAAX and cells that did not express the latter as controls ( Fig. 4e ). The results indicated that the Magnet-based photoactivatable PI3K rapidly generated PI(3,4,5)P 3 upon blue light irradiation; thus, this method induced PI(3,4,5)P 3 -dependent morphological changes in the PM. We conducted spatially and temporally confined optical control of PI3K with pMagFast2(3x). COS-7 cells were expressed with iSH2-pMagFast2(3x)-iRFP and nMagHigh1-CAAX with Lifeact-mCherry. After focal irradiation of the cells, directed lamellipodia were rapidly generated around the irradiated portion of the PM ( Fig. 4f , center and Fig. 4g , upper). Membrane retraction was observed on the opposite side of the irradiated-cell edge, as seen in the naturally occurring rear side of migrating cells ( Fig. 4f , center and Fig. 4g , lower). These data showed that the asymmetric activation of pMagFast2(3x)-based photoactivatable PI3K induced cell polarity in single cells. When the irradiation was shifted from the initial area to the opposite side of the same cell, a reversal of the cell polarity was observed ( Fig. 4f , right and Fig. 4g ). Treatment of the cells with LY294002 fully blocked the morphological change induced by focal irradiation with blue light ( Fig. 4h,i ). Thus, photoactivatable PI3K using pMagFast2(3x) allowed for the rapid and reversible generation of PI(3,4,5)P 3 and induced lamellipodia formation at high spatiotemporal patterns. We also developed photoactivatable actuators for a small GTPase Rac1 (ref. 27 ) using pMagFast2(3x) ( Supplementary Fig. 6 ). In response to global irradiation with blue light, pMagFast2(3x)-based photoactivatable Rac1 induced a striking morphological change in the cells that led to the global formation of lamellipodia and membrane ruffles ( Supplementary Fig. 7a ). The expanded area of the cells was quantitatively analysed ( Supplementary Fig. 7e ). The observed morphological change in the PM was completely blocked by a potent Rac1-specific GEF inhibitor ( Supplementary Fig. 7b,e ). We also examined that cells not expressing both Tiam1-pMagFast2(3x)-iRFP and nMagHigh1-CAAX and those not expressing the latter did not change their morphology before and after blue light irradiation ( Supplementary Fig. 7c–e ). The results of pMagFast2(3x)-based photoactivatable PI3K and Rac1 demonstrated that the present photoswitches provide a robust tool to spatially and temporally control a variety of cellular proteins and related cellular functions with light. We have completed a multi-directional engineering of the fungal photoreceptor VVD and created novel photoswitches named Magnets ( Supplementary Fig. 8 ). First, we modified the dimer interface of VVD to prevent unwanted homodimerization and selectively induce heterodimerization. As a result, we generated a pair of two distinct VVD variants that recognize each other based on electrostatic interactions. Next, additional engineering of the cofactor-binding domain was performed to tune the switch-off kinetics of the heterodimer. We generated two contrasting variants, including one with an ~250-fold accelerated switch-off kinetics but diminished dimerization efficiencies and one variant with a 17-fold enhanced dimerization efficiency but slower switch-off kinetics. We have solved this trade-off problem by pairing the two contrasting variants to create the present photoswitches that showed substantially enhanced dimerization efficiencies and accelerated switch-off kinetics. We showed that pMagFast2–nMagHigh1 exhibited switch-off kinetics with a half-life t 1/2 of 6.8 s in mammalian cells. This is substantially faster than any other conventional dimerization-based blue photoswitches reported for optogenetic applications in living cells, including CRY2–CIB1 ( t 1/2 , ~5.5 min) [7] , FKF1–GI ( t 1/2 , >90 min) [6] and TULIPs ( t 1/2 , 2.8 min) [11] . In addition to the present fast photoswitches, we also have developed photoswitches with slow switch-off kinetics, such as pMag–nMagHigh1 ( t 1/2 , 2.1 h; rate constant, 9.3 × 10 −5 ) and pMagHigh1–nMagHigh1 ( t 1/2 , 4.7 h). While the fast photoswitches provide a powerful tool for spatially and temporally confined optical control of protein activities in the cells, the slow photoswitches require only a one-shot irradiation to act as a continuously active optogenetic tool. The slow photoswitches could be used to avoid some unwanted side effects caused by continuous irradiation, such as phototoxicity and unfocused activation owing to sample drift. Recently, methods to improve switch-off kinetics of blue light photoreceptors have been developed using bacterial or yeast colonies-based high throughput screening systems [28] , [29] . These screening methods can help to further accelerate or decelerate the switch-off kinetics of the present photoswitches. In addition to the tunable property of the switch-off kinetics, which ranged from seconds to hours, Magnets consist of two photosensory units. Thus, Magnets are only switched on when both the photosensory units are simultaneously activated, similar to an AND-logic gate. In contrast, existing photoswitches consist of photosensory units and binder units [1] that can only be switched on if the photosensory units are activated. This is because the binder units are always active. The synergistic activation property of Magnets contributes to their extremely low dimerization activity in the dark state. The present photoswitches, created by re-engineering the nature of a natural photoreceptor, provide new opportunities for the optogenetic control of a wide variety of cellular proteins and related cellular functions. Materials We used a N-terminal truncated version (residues 37–186, 17.1 kDa) of VVD because it is more stable than the full length VVD (residues 1–186, 21.3 kDa) [14] . cDNAs encoding VVD and its variants with codons optimized for mammalian expression were synthesized by Invitrogen (Carlsbad, CA, USA) and DNA2.0 (Menlo Park, CA, USA). cDNA encoding iRFP with codons optimized for mammalian expression was synthesized by GenScript (Piscataway, NJ, USA). cDNA encoding mouse Tiam1 was obtained from Addgene (Cambridge, MA, USA). cDNA encoding humanized monomeric Kikume Green-Red (mKikGR) [30] was obtained from MBL (Nagoya, Japan). The pharmacological inhibitor of PI3kinase (LY294002) was purchased from Sigma Chemical (St. Louis, MO, USA). The pharmacological inhibitor of Rac1 (Rac1 Inhibitor) was purchased from Wako (Osaka, Japan). All cloning enzymes were obtained from Takara Biomedical (Tokyo, Japan) and used according to the manufacturer’s instructions. Plasmid construction and mutagenesis The mutagenesis of VVD was performed with an overlap extension technique and Multi Site-Directed Mutagenesis Kit (MBL) according to the manufacturer’s instructions [31] , [32] . The obtained mutants were sequenced with an ABI310 genetic analyzer (Applied Biosystems, Foster City, CA, USA): pMag, I52R/M55R; pMagFast1, I52R/M55R/I85V; pMagFast2, I52R/M55R/I74V/I85V; pMagHigh1, I52R/M55R/M135I/M165I; nMag, I52D/M55G; nMagFast1, I52D/M55G/I85V; nMagFast2, I52D/M55G/I74V/I85V; and nMagHigh1, I52D/M55G/M135I/M165I. All of the cDNAs constructed for characterization of the present photoswitches are listed in Supplementary Figs 1a, 9 and 10 . All of primers for the site-directed mutagenesis of VVD are listed in Supplementary Table 1 . Cell culture COS-7 and NIH3T3 cells (American Type Culture Collection (ATCC)) were cultured at 37 °C under 5% CO 2 in Dulbecco’s Modified Eagle Medium (DMEM; Invitrogen) supplemented with 10% fetal bovine serum (GIBCO, Carlsbad, CA, USA), 100 unit ml −1 penicillin and 100 μg ml −1 of streptomycin (GIBCO). Bioluminescence assay For the screening of VVD variants, COS-7 cells were plated at ~2.0 × 10 4 cells per well in 96-well black-walled plates (Thermo Fisher Scientific, Walthman, MA, USA) and cultured for 24 h at 37 °C in 5% CO 2 . The cells were then transfected with Lipofectamine 2000 reagent (Invitrogen) according to the manufacturer’s protocol. cDNAs encoding Nfluc-X and X(Y)-Cfluc (X and Y stand for VVD variants) were transfected at a 1:1 ratio. The total amount of DNA was 0.4 μg per well. Twenty-four hours after transfection, the culture medium was replaced with 100 μl of a luciferase assay reagent (Promega, Madison, WI, USA) containing D -luciferin as a substrate. The luciferase assay reagent was prepared by adding 5 ml of Hanks' Balanced Salt Solution (HBSS, Grand Island Biological , Grand Island, NY, USA) to one vial of the lyophilized luciferase assay substrate (Promega). After cells were treated with the luciferase assay reagent for 1 h at room temperature, bioluminescence measurements were performed for 10 s at room temperature using a Centro XS 3 LB 960 plate-reading luminometer (Berthold Technologies, Bad Wildbad, Germany). Blue light irradiation was performed using a LED light source (470 nm±20 nm; CCS, Kyoto, Japan). Irradiation time and the intensity of blue light were 30 s and 3 mW cm −2 , respectively. For the dissociation kinetics analysis of the VVD variants, COS-7 cells were plated at ~10 × 10 4 cells per well in a 24-well plate (Nunc, Roskilde, Denmark) and cultured for 24 h at 37 °C in 5% CO 2 . The cells were then transfected with Lipofectamine 2000 reagent. cDNAs encoding Nfluc-X and X(Y)-Cfluc were transfected at a 1:1 ratio. The total amount of DNA was 0.8 μg per well. Twenty-four hours after transfection, the culture medium was replaced with 500 μl of the luciferase assay reagent. The cells were scraped and collected in Röhren polystyrene tubes (Sarstedt, Nümbrecht, Germany). After cells were treated with the luciferase assay reagent for 1 h at room temperature, the sample tube was placed into a Lumat LB 9507 single-tube luminometer (Berthold Technologies), and bioluminescence measurements were performed using the luminometer. The bioluminescence signals were integrated over 1 s at room temperature and plotted every 1 s. To expose the cells to blue light, we stopped the measurement of bioluminescence intensity and removed the sample tube from the luminometer. We then irradiated the sample tube with blue light by using an LED light source (470±20 nm, 3 mW cm −2 , 30 s) and immediately placed the sample tube back into the luminometer to resume the bioluminescence measurement. The time elapsing from the shut-off of blue light irradiation to the resuming of the bioluminescence measurement was less than 1 s. We fitted the dissociation curves to mono-exponential functions to determine the half-life t 1/2 . Live cell imaging Glass-bottomed dishes (Iwaki Glass, Chiba, Japan) were coated with 25 μg ml −1 of human fibronectin (BD Biosciences, Franklin Lakes, NJ, USA) at room temperature for 1 h and then washed twice with 2 ml of Milli-Q water. To conduct the PM-translocation assay of the photoswitches using TIRF imaging, COS-7 cells were plated at 1.0 × 10 4 cells per dish on glass-bottomed dishes and cultured for 24 h at 37 °C in 5% CO 2 . The cells were transfected with cDNAs encoding pMag(3x)-mCherry and nMagHigh1-mKikGR-CAAX at a 1:1 ratio using X-tremeGENE 9 reagent at 37 °C. The total amount of DNA was 1 μg per dish. Twenty-four hours after transfection, the medium was replaced by a DMEM culture medium supplemented with 10% FBS. The cells were maintained for 18–26 h at 28 °C. Before imaging, the culture medium was replaced with HBSS containing 25 mM HEPES. Imaging was performed at room temperature with a 100 × oil objective on the stage of an ECLIPSE T i TIRF microscope (Nikon, Tokyo, Japan). Fluorescence images of mCherry were taken using an optically pumped semiconductor laser at 561 nm (Coherent, CA, USA). Blue light irradiation was conducted using an optically pumped semiconductor laser (488 nm) at 1 mW for 50 ms. For confocal imaging of the PM-translocation of the photoswitches, NIH3T3 cells were plated at 2.0 × 10 4 cells per dish on glass-bottomed dishes and cultured for 24 h at 37 °C in 5% CO 2 . The cells were transfected with cDNAs encoding pMagFast2(3x)-iRFP and nMagHigh1-EGFP-CAAX at a 1:7 ratio using Lipofectamine 2000 reagent at 37 °C. The total amount of DNA was 0.4 μg per dish. Twenty-four hours after transfection, the medium was replaced by a DMEM culture medium supplemented with 10% FBS. The cells were maintained for 18–26 h at 28 °C. Before imaging, the culture medium was replaced with HBSS containing 25 mM HEPES. Imaging was conducted at 37 °C with a 63 × oil objective on the stage of a LSM 710 confocal laser-scanning microscope (Carl Zeiss, Jena, Germany) with a heated stage adaptor (Tokai Hit , Fujinomiya, Japan). Fluorescence images of EGFP and iRFP were taken using a Multi-line Argon laser (514 nm) and a HeNe laser (633 nm), respectively. Blue light irradiation was completed with a Multi-line Argon laser (488 nm) at 2 mW. To examine Magnet-based photoactivatable PI3K, NIH3T3 cells were plated at 0.8 × 10 4 cells per dish on glass-bottomed dishes and cultured for 24 h at 37 °C in 5% CO 2 . The cells were transfected with cDNAs encoding iSH2-pMag(3x)-iRFP, nMagHigh1-EGFP-CAAX and AktPH-mCherry at a 1:37:2 ratio using Lipofectamine 2000 reagent. The total amount of DNA was 0.4 μg per dish. Twenty-four hours after transfection, the medium was replaced by a DMEM culture medium supplemented with 10% FBS. The cells were maintained for 24–30 h at 28 °C. Before imaging, the cells were incubated in serum-free DMEM culture medium for at least 3 h. Imaging was conducted at room temperature with a 63 × oil objective on the stage of a LSM 710 confocal laser-scanning microscope. Fluorescence images of EGFP, mCherry and iRFP were taken using a Multi-line Argon laser (514 nm) and a HeNe laser (543 nm, 633 nm), respectively. Blue light irradiation was completed with a Multi-line Argon laser (488 nm) at 2 mW. To observe morphological changes in the PM using Magnet-based photoactivatable PI3K and Rac1, COS-7 cells were plated at 0.2 × 10 4 cells per dish on glass-bottomed dishes coated with fibronectin. The cells were transfected with iSH2-pMag(3x)-iRFP or iSH2-pMagFast2(3x)-iRFP or Tiam1-pMagFast2(3x)-iRFP, nMagHigh1-EGFP-CAAX and Lifeact-mCherry at a 1:27:2 ratio using X-tremeGENE 9 reagent. The total amount of DNA was 0.4 μg per dish. Blue light irradiation was completed with a Multi-line Argon laser (488 nm) at 2 or 0.2 mW. Quantitative analysis of expanded cell area The area of COS-7 cells expressing Lifeact-mCherry was analysed based on the fluorescence intensity of mCherry using Image-J software. The expanded areas were calculated by subtracting cell areas before blue light irradiation from those after 20 min of irradiation. Statistical analysis Statistical significance ( P value) was determined using a two-tailed Student’s t -test. Curve fitting We fitted the switch-on/off kinetics of bioluminescence and fluorescence of Magnets to the following mono-exponential equation using the online curve-fitting tool at http://zunzun.com : Y = Ae − kt + B , where Y represents fluorescence intensity at time t , A and B are parameters, and k represents the rate constant. The half-life, t 1/2 , was determined using the following equation: t 1/2 =ln2 k − 1 . How to cite this article: Kawano, F. et al . Engineered pairs of distinct photoswitches for optogenetic control of cellular proteins. Nat. Commun. 6:6256 doi: 10.1038/ncomms7256 (2015).